Molecular stratification of endometrioid ovarian carcinoma predicts clinical outcome Endometrioid ovarian carcinoma (EnOC) demonstrates substantial clinical and molecular heterogeneity. Here, we report whole exome sequencing of 112 EnOC cases following rigorous pathological assessment. We detect a high frequency of mutation in CTNNB1 (43%), PIK3CA (43%), ARID1A (36%), PTEN (29%), KRAS (26%), TP53 (26%) and SOX8 (19%), a recurrently-mutated gene previously unreported in EnOC. POLE and mismatch repair protein-encoding genes were mutated at lower frequency (6%, 18%) with significant co-occurrence. A molecular taxonomy is constructed, identifying clinically distinct EnOC subtypes: cases with TP53 mutation demonstrate greater genomic complexity, are commonly FIGO stage III/IV at diagnosis (48%), are frequently incompletely debulked (44%) and demonstrate inferior survival; conversely, cases with CTNNB1 mutation, which is mutually exclusive with TP53 mutation, demonstrate low genomic complexity and excellent clinical outcome, and are predominantly stage I/II at diagnosis (89%) and completely resected (87%). Moreover, we identify the WNT, MAPK/RAS and PI3K pathways as good candidate targets for molecular therapeutics in EnOC. Ovarian carcinomas (OC) are a heterogeneous group of malignancies comprising five core histological types, each with distinct pathological characteristics, molecular landscapes and clinical behaviour [1] , [2] . Endometrioid OC (EnOC) accounts for approximately 10% of all OC, with the majority of cases diagnosed as low grade, early stage disease with excellent clinical outcome [3] , [4] , [5] . Currently, the management of EnOC follows the historic one-size-fits-all approach of aggressive cytoreductive surgery with adjuvant platinum–taxane chemotherapy for patients with disease that has progressed beyond the ovary/fallopian tube. By contrast, routine molecular stratification of care is emerging in other OC types, most notably with the advent of poly(adenosine diphosphate-ribose) polymerase (PARP) inhibitor therapy [6] , [7] . Targeted sequencing approaches have identified PTEN, ARID1A, PIK3CA, KRAS, CTNNB1 , and genes encoding mismatch repair (MMR) proteins as frequently mutated in relatively small cohorts of EnOC [8] , [9] , [10] , reminiscent of endometrioid endometrial carcinoma (EnEC) [11] , with a TP53 mutation ( TP53 m) rate markedly lower than their high grade serous OC (HGSOC) counterparts [12] . Recent whole genome sequencing of a small EnOC case series has recapitulated these findings and identified a small proportion of EnOC with extensive copy number alterations (CNAs) more akin to the genomic instability demonstrated by HGSOC [13] . The majority of EnOC are believed to arise from endometriosis [1] , and most grade 1 and 2 (low grade) EnOC display a classical immunohistochemical (IHC) profile comprising Wilms’ tumour 1 (WT1) negativity, wild-type tumour protein p53 (p53) expression, and oestrogen receptor (ER) positivity [4] . These classical low grade EnOC bear close histological resemblance to EnEC [14] . Grade 3 (high grade) EnOC can be challenging to differentiate from HGSOC on the basis of morphology alone [4] , [14] . In particular, HGSOC demonstrating the solid, pseudo-endometrioid and/or transitional-cell-like (SET) histological pattern, which may be associated with BRCA1 mutations [15] , represent a population easily misclassified as EnOC. Indeed, it is now recognised that many historically diagnosed high grade EnOC in fact represent HGSOC, supported by transcriptomic studies demonstrating that a proportion of high grade EnOC cluster with HGSOC [16] , [17] , [18] , [19] . As such, true high grade EnOC are increasingly rare, representing only around 5–19 % of EnOC cases [4] , [9] , [20] , [21] ; these patients reportedly experience poor clinical outcome, in contrast to their low grade counterparts [3] , [21] . To date, the overwhelming body of clinical and molecular EnOC characterisation has been confounded by the inclusion of historically misclassified HGSOC. Mutational analyses performed by more recent studies have either been applied to low grade EnOC alone [22] , or lack information on grade or diagnostic criteria used [8] , [23] and have ubiquitously analysed small patient cohorts with insufficient power to confidently correlate molecular events with patient outcome. As a result, the molecular landscape of EnOC, in particular high grade EnOC, is poorly defined. WT1 IHC is a useful tool to discriminate high grade EnOC (WT1 negative) from HGSOC (WT1 positive), reducing interobserver variation [16] , [20] , [24] , [25] , [26] , [27] . Here, we perform molecular characterisation of contemporarily defined EnOC with the use of IHC for WT1. We perform whole exome sequencing (WES) to define the genomic landscape of EnOC, including high grade EnOC, in a sizeable cohort of otherwise unselected patients. We identify subtypes of EnOC that display distinct clinical behaviour, constructing a step-wise taxonomy for EnOC classification based on mutation status of TP53 and CTNNB1 . TP53 m cases, characterised by greater genomic complexity and frequent CNA events, demonstrate poor survival; conversely, cases with CTNNB1 mutation ( CTNNB1 m)—which occurs mutually exclusively with TP53 m—are of low genomic complexity with few CNA events and demonstrate excellent long-term survival. The remaining cases represent a subtype with intermediate prognosis. Clinical characteristics Of 289 historically diagnosed EnOC cases identified with available tumour material, 112 WT1 negative cases were characterised by WES following rigorous pathology review (Fig. 1 ). 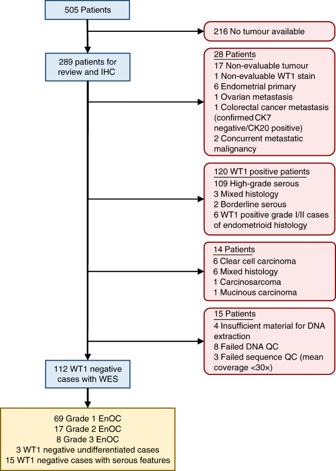Fig. 1: Flow diagram identifying endometrioid ovarian carcinoma cases for whole exome sequencing. IHC immunohistochemistry, WES whole exome sequencing, EnOC endometrioid ovarian carcinoma, WT1 Wilms’ tumour 1, QC quality control. The clinicopathological characteristics of these patients are shown in Table 1 . The majority of patients presented with stage I or II disease (78.2%, 86 of 110 evaluable cases; 2 unknown stage); 27 stage I/II cases received no adjuvant chemotherapy. Nineteen cases (17.0%) had concurrent endometrial cancer diagnosis. The median follow-up time was 13.0 years. Five-year disease-specific survival (DSS) and progression-free survival (PFS) across the cohort was 72.8% (95% CI 64.8–81.8%) and 68.5% (95% CI 60.2–77.9%). Fig. 1: Flow diagram identifying endometrioid ovarian carcinoma cases for whole exome sequencing. IHC immunohistochemistry, WES whole exome sequencing, EnOC endometrioid ovarian carcinoma, WT1 Wilms’ tumour 1, QC quality control. Full size image Table 1 Clinical characteristics of the 112 endometrioid ovarian carcinoma cases. Full size table Genomic landscape of endometrioid ovarian carcinoma The most commonly mutated genes included CTNNB1 (48 cases, 42.9%), PIK3CA (48 cases, 42.9%), ARID1A (40 cases, 35.7%), PTEN (33 cases, 29.5%), KRAS (29 cases, 25.9%), and TP53 (29 cases, 25.9%) (Supplementary Fig. 1 ). Unsupervised hierarchical clustering across the 50 most commonly mutated genes revealed mutation of TP53 and CTNNB1 ( TP53 m and CTNNB1 m) as the most prominent stratifying events (Fig. 2 and Supplementary Fig. 2 ). TP53 m and CTNNB1 m were largely mutually exclusive (Fig. 3a ), with significant depletion of CTNNB1 m in the TP53 m group ( P < 0.001; co-occurrence in one case, 0.9%). The CTNNB1 m rate in the TP53 wild-type ( TP53 wt) group was 56.6% (47 of 83 TP53 wt cases). Fig. 2: Unsupervised clustering of endometrioid ovarian carcinomas by patterns of mutation. Product-moment correlation scores between samples were calculated using binary matrices representing the status of most frequently mutated genes (1 = mutant, 0 = wild-type), yielding a matrix of quantified genomic correlation. These data were subject to hierarchical clustering using Euclidean distance and Ward’s linkage. Bars denote mutation in CTNNB1 and TP53 . Full size image Fig. 3: Genomic characterisation of endometrioid ovarian carcinoma (EnOC). a Whole exome sequencing identifies three major genomic subtypes of endometrioid ovarian carcinoma based on TP53 and CTNNB1 mutation status. Molecular signatures for each tumour are plotted as the fraction of transversions and transitions. Mutations are displayed as an oncoplot. Grey denotes no mutation. Upper plot shows the six most frequently mutated genes; lower plot shows select genes of interest. b Lollipop plots of five common gene targets of mutation. c Mismatch repair (MMR) mutations across cases. d Relationship between tumour mutational burden (TMB) and mutations in POLE and/or MMR genes. Ti transition, tv transversion, MSI microsatellite instability, RD residual disease. Full size image Mutation of SOX8 , a gene target of mutational disruption previously unreported at high frequency in EnOC, was also identified as a common event (21 cases, 18.8%), alongside other targets of mutation (Fig. 3a and Supplementary Figs. 1 , 3A ). There was significant enrichment of SOX8 m in the TP53 m group (10/29, 34.5% SOX8 m in the TP53 m group vs. 11/83, 13.3% SOX8 m in the TP53 wt group; P = 0.025). Events in other genes previously reported as mutated in EnOC or endometrial cancer were identified at lower frequency, including FBXW7 m (14 cases, 12.5%), KMT2D/MLL3 m (12 cases, 10.7%) , BRCA1/2 m (14 cases, 12.5%) (Supplementary Table 1 ), PIK3R1 m (10 cases, 8.9%), MTOR m (7 cases, 6.3%), POLE m (7 cases, 6.3%) (Supplementary Fig. 3B ), APC (6 cases, 5.4%) and PPP2R1A m (4 cases, 3.6%) (Fig. 3a and Supplementary Fig. 1 ). BRCA1 / 2 m cases demonstrated a high rate of TP53 m (57.1%, 8 of 14 cases) and a high rate of mutation in genes previously reported in EnOC (71.4%, 10 of 14 cases with mutations in ARID1A , CTNNB1 , PTEN , PIK3CA , KRAS , or genes encoding mismatch repair proteins). Pathway analysis identified a large number of mutations across four major oncogenic pathways: PI3K-AKT, WNT, RAS, and NOTCH (Supplementary Fig. 4 ). Tumour mutational burden (TMB) and microsatellite instability (MSI) A median of 78 variants were detected per sample (range 42–2894) (Supplementary Figs. 5 , 6A ). Ten cases (8.9%) were considered hypermutated (>250 mutations per sample) and 3 (2.7%) were considered ultramutated (>1000 mutations) (Fig. 3a ). Overall analysis of TMB against TCGA derived datasets places EnOC alongside HGSOC (median TMB = 72), colonic adenocarcinoma (median TMB = 76) and EnEC (median TMB = 78) (Supplementary Fig. 6B ). Mutations in one or more genes encoding MMR proteins were identified in 20 cases (17.9%) (Fig. 3c ), most commonly in MSH3, MSH6 , MLH3 or MSH4 . The majority of MMR-mutant (MMRm) tumours were TP53 wt (18/20 cases, 90.0%). High impact MMRm (frameshifting InDels, nonsense or splice site mutations) were associated with significantly higher MSI scores compared to those containing missense MMRm (median 236 vs. 142.5, P < 0.001) and MMRwt samples (median 236 vs. 162, P < 0.001) (Fig. 3a and Supplementary Fig. 7 ). There was no significant difference in MSI score between MMRwt cases and those with missense MMRm ( P = 0.194). POLE m commonly occured over a hotspot within the exonuclease domain (42.9%, 3 of 7 POLE m cases) (Supplementary Fig. 3B ). There was a high frequency of concurrent POLE m and MMRm (five of seven POLE m cases, 71.4%), with significant enrichment for MMRm within the POLE m versus POLE wt group (71.4%, 5/7 vs. 14.3%, 15/105, P = 0.002). Together, the POLE m and high impact MMRm cases accounted for the majority of high TMB cases (Fig. 3d ). Cases with concurrent POLE m and MMRm accounted for all three ultramutated tumours; 8 of the 10 (80.0%) hypermutated tumours contained either POLE m or high impact MMRm. Mutational spectrum in endometrioid ovarian carcinoma We observed a bias towards C>T and C>A transversion and transition molecular signatures across the 112 EnOC cases (Fig. 3a ). A shift in signatures was observed in samples harbouring POLE m, with a greater proportion of T>G changes, and depletion of C>G and T>A substitutions in this population (Supplementary Fig. 8 ). Tumour genomic complexity and copy number alterations Distribution of per-sample global variant allele frequency (VAF) density and calculation of mutant-allele tumour heterogeneity (MATH) score across the 112 EnOC cases was used to infer tumour genomic complexity (Fig. 4 ). TP53 wt tumours were predominantly low complexity, demonstrating lower MATH scores (median 27.5 vs. 54.7, P < 0.001) (Fig. 4b, c and Supplementary Fig. 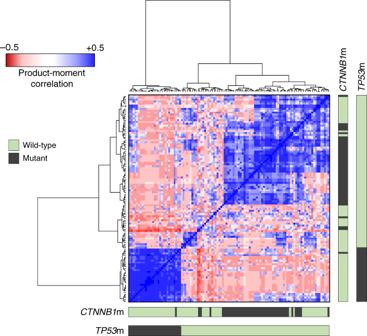Fig. 2: Unsupervised clustering of endometrioid ovarian carcinomas by patterns of mutation. Product-moment correlation scores between samples were calculated using binary matrices representing the status of most frequently mutated genes (1 = mutant, 0 = wild-type), yielding a matrix of quantified genomic correlation. These data were subject to hierarchical clustering using Euclidean distance and Ward’s linkage. Bars denote mutation inCTNNB1andTP53. 9A ) and fewer discrete VAF peaks ( P < 0.001) (Supplementary Table 2 ) compared to TP53 m cases. Fig. 4: Genomic complexity of endometrioid ovarian carcinomas (EnOC). a Representative examples of variant allele frequency density plots for a high complexity tumour (left), intermediate complexity tumour (centre) and low complexity tumour (right). Variant allele frequency (VAF) clusters are shown and summarised within box plots above the density plot; boxes represent the 1st to 3rd quartile, with the median labelled as the central line, and whiskers extend to the data range from 1st and 3rd quartile +/−1.5 times the interquartile range. b Mutant-allele tumour heterogeneity (MATH) genomic complexity scores across all 112 endometrioid ovarian carcinoma (EnOC) cases, ranked high to low. c MATH genomic complexity scores across the three EnOC subtypes. Comparisons were made using the two-sided Mann–Whitney U -test without adjustment for multiple testing ( P < 0.0001 and P = 0.0353). m mutant, wt wild-type. Full size image Analysis of CNA events across samples revealed differential CNA burden across molecular subgroups defined by TP53 m and CTNNB1 m status, with TP53 m cases harbouring greater CNA burden compared to TP53 wt tumours ( P < 0.0001) (Supplementary Figs. 9B , 10A , B ). The most frequent CNA events across the cohort were gain of ZNF43 (30 cases, 26.8%), RABA1C (24 cases, 21.4%) and AMY1C (23 cases, 20.5%), and loss of PKNOX1 (42 cases, 37.5%), CEP68 (29 cases, 25.9%) and GLB1L (20 cases, 17.9%) (Supplementary Fig. 10C ). CNA events were also identified over genes that were frequent targets of mutational disruption (Supplementary Fig. 10D ). Molecular events define clinically distinct disease subtypes TP53 m cases demonstrated significantly inferior DSS upon univariable analysis (HR = 4.43, 95% CI 2.27–8.64, Bonferroni-adjusted P < 0.001) (Supplementary Figs. 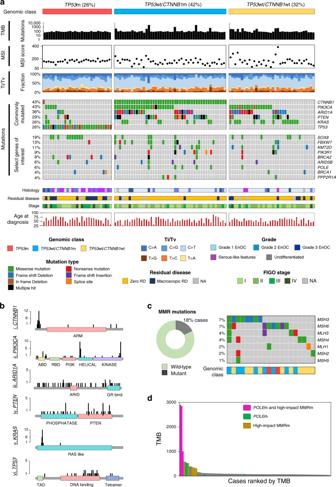Fig. 3: Genomic characterisation of endometrioid ovarian carcinoma (EnOC). aWhole exome sequencing identifies three major genomic subtypes of endometrioid ovarian carcinoma based onTP53andCTNNB1mutation status. Molecular signatures for each tumour are plotted as the fraction of transversions and transitions. Mutations are displayed as an oncoplot. Grey denotes no mutation. Upper plot shows the six most frequently mutated genes; lower plot shows select genes of interest.bLollipop plots of five common gene targets of mutation.cMismatch repair (MMR) mutations across cases.dRelationship between tumour mutational burden (TMB) and mutations inPOLEand/or MMR genes. Ti transition, tv transversion, MSI microsatellite instability,RDresidual disease. 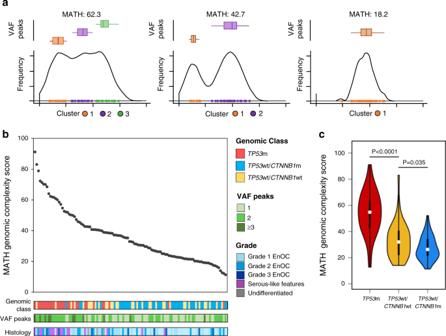Fig. 4: Genomic complexity of endometrioid ovarian carcinomas (EnOC). aRepresentative examples of variant allele frequency density plots for a high complexity tumour (left), intermediate complexity tumour (centre) and low complexity tumour (right). Variant allele frequency (VAF) clusters are shown and summarised within box plots above the density plot; boxes represent the 1st to 3rd quartile, with the median labelled as the central line, and whiskers extend to the data range from 1st and 3rd quartile +/−1.5 times the interquartile range.bMutant-allele tumour heterogeneity (MATH) genomic complexity scores across all 112 endometrioid ovarian carcinoma (EnOC) cases, ranked high to low.cMATH genomic complexity scores across the three EnOC subtypes. Comparisons were made using the two-sided Mann–WhitneyU-test without adjustment for multiple testing (P< 0.0001 andP= 0.0353). m mutant, wt wild-type. 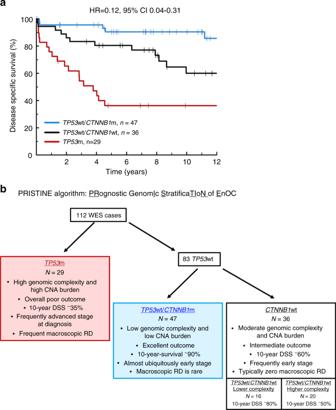Fig. 5: Genomic subtypes of endometrioid ovarian carcinoma demonstrate distinct clinical behaviour. aDisease-specific survival based onTP53m andCTNNB1m status; labelled hazard ratio represents comparison of theTP53wt/CTNNB1m group with theTP53m group. HR forTP53wt/CTNNB1wt vs.TP53m = 0.37, 95% CI 0.18–78; HR forTP53wt/CTNNB1m vs.TP53wt/CTNNB1wt = 0.31, 95% CI 0.11–0.88.bSummary of the PRISTINE algorithm for molecular subtyping in endometrioid ovarian carcinoma. m mutant, wt wild-type, RD residual disease, WES whole exome sequencing, DSS disease-specific survival. 11A , 12A and Supplementary Table 3 ), were more likely to be diagnosed at advanced stage (14 of 29 evaluable cases, 48.3% stage III/IV vs. 10 of 81, 12.3%; P < 0.001) (Supplementary Table 4 ), less likely to be successfully resected to zero macroscopic residual disease (RD) (44.4%, 12 of 27 evaluable cases with macroscopic RD after surgical debulking vs. 14.1%, 11 of 78; P = 0.003), and demonstrated a trend for greater age at diagnosis which did not meet statistical significance (median 61 vs. 57 years, P = 0.063). Multivariable analysis accounting for patient age, stage at diagnosis, and extent of RD following primary cytoreduction identified TP53 m as independently associated with shorter DSS ( P = 0.031) (Supplementary Tables 5 , 6 ). The TP53 m group demonstrated significant depletion of cases with concurrent endometrial cancer diagnosis (3.4%, 1 of 29 TP53 m vs. 21.7%, 18 of 83 TP53 wt, P = 0.023). The median DSS and PFS for TP53 m cases were 3.78 and 1.54 years, respectively. By contrast, cases with CTNNB1 m were overwhelmingly stage I/II at diagnosis (89.1%, 41 of 46 evaluable cases) and debulked to zero macroscopic RD (87.0%, 42 of 46 evaluable cases), with markedly favourable outcome (HR for DSS = 0.23, 95% CI 0.10–0.56, Bonferroni-adjusted P = 0.010) (Supplementary Figs. 11B , 12B and Supplementary Table 3 ) which was significant upon multivariable analysis ( P = 0.017) (Supplementary Tables 7 , 8 ). CTNNB1 m was significantly associated with favourable outcome specifically in the context of TP53 wt cases (HR for DSS = 0.31, 95% CI 0.11–0.88) (Fig. 5a ), and TP53 wt/ CTNNB1 m cases were less genomically complex vs. their TP53 wt/ CTNNB1 wt counterparts (median MATH score 26.3 vs. 31.9, P = 0.035) with fewer CNA events ( P = 0.042) (Fig. 4c and Supplementary Fig. 10B ). The DSS difference between genomic subgroups defined by combined TP53 m and CTNNB1 m status was maintained upon exclusion of cases with concurrent endometrial carcinoma ( P < 0.001) (Supplementary Fig. 13 ) and upon exclusion of cases demonstrating TP53 m in the absence of endometrioid-associated mutations ( P < 0.001) (Supplementary Fig. 14 ). Fig. 5: Genomic subtypes of endometrioid ovarian carcinoma demonstrate distinct clinical behaviour. a Disease-specific survival based on TP53 m and CTNNB1 m status; labelled hazard ratio represents comparison of the TP53 wt/ CTNNB1 m group with the TP53 m group. HR for TP53 wt/ CTNNB1 wt vs. TP53 m = 0.37, 95% CI 0.18–78; HR for TP53 wt/ CTNNB1 m vs. TP53 wt/ CTNNB1 wt = 0.31, 95% CI 0.11–0.88. b Summary of the PRISTINE algorithm for molecular subtyping in endometrioid ovarian carcinoma. m mutant, wt wild-type, RD residual disease, WES whole exome sequencing, DSS disease-specific survival. Full size image POLE m EnOC cases did not demonstrate an obvious exceptional 5-year survival pattern akin to that reported in POLE m endometrial carcinomas, and did not demonstrate prolonged DSS vs. POLE wt patients (5-year DSS 85.7%; P = 0.337 vs. POLE wt) (Supplementary Table 3 ), although case numbers were extremely low ( n = 7). Greater tumour complexity was associated with inferior survival when defined by the number of VAF peaks ( P = 0.020 for DSS) or continuous MATH score ( P < 0.001 for DSS) (Supplementary Table 9 ). Exploratory analysis to determine whether the outcome of TP53 wt/ CTNNB1 wt cases could be further resolved by genomic complexity identified that low complexity TP53 wt/ CTNNB1 wt cases (MATH score ≤ median MATH score in EnOCs with a single VAF peak) demonstrated relatively favourable outcome (10-year DSS 77.0%) (Supplementary Fig. 15 ), while their more genomically complex counterparts demonstrated intermediate prognosis (10-year DSS 48.7%); however, this difference did not reach statistical significance and case numbers were limited. Together, these data support a clinically meaningful classification system driven TP53 m and CTNNB1 m status in a step-wise fashion, which we present here as the PRISTINE algorithm: PRognostic genomIc StratificaTIoN of EnOC (Fig. 5b ). Genomic complexity may represent a potential tool to further discriminate outcome in these subtypes. Utility of immunohistochemistry to identify disease subtypes IHC for p53 and β-catenin, the protein products of TP53 and CTNNB1 , was able to identify subgroups of EnOC with differential DSS ( P < 0.001 and P = 0.045) (Supplementary Fig. 16A, B ). Combined use of these markers to recapitulate the PRISTINE algorithm identified patient groups with differential DSS akin to those defined by genomic data ( P < 0.001) (Supplementary Fig. 16C ). However, aberrant β-catenin expression (βcat-aberrant) resolved outcome less well in those with wild-type p53 protein expression (p53-wt) compared to CTNNB1 m status in the TP53 wt group (Fig. 5a ), likely owing to the suboptimal sensitivity of β-catenin IHC for CTNNB1 m (Supplementary Fig. 16B ). The molecular landscape of EnOC is poorly defined, particularly in high grade cases, due to under-investigation and historic misclassification of HGSOC as high grade EnOC in older studies. WT1 negativity has emerged as an important discriminator of high grade EnOC from HGSOC, which displays morphological similarities [4] , [24] , [25] , [26] , [27] . To our knowledge, this is the largest report of genomically characterised EnOC to date, utilising routine WT1 IHC to exclude pseudo-endometrioid HGSOC that have contaminated previous studies of this cancer type. In line with previous sequencing studies in small cohorts of EnOC, we identified a high mutation rate of genes known to be perturbed in EnEC, the most frequent of which were CTNNB1 , PIK3CA , PTEN , ARID1A , KRAS , and TP53 [8] , [11] , [22] , [28] , [29] . Our EnOC cohort demonstrated a similar rate of TP53 m to the TCGA study of EnEC [11] ; by contrast, the mutation rate of PTEN was lower. We demonstrate that EnOC tumours contain a moderate TMB with respect to other cancer types, with a small proportion hyper-mutated or ultra-mutated in nature (11.6%). MMR deficiency due to mutations or methylation in MMR protein-encoding genes results in MSI, and loss of MMR protein expression has previously been demonstrated in approximately 7–14% of EnOC [30] , [31] , [32] , [33] , [34] . As in EnEC, we identify a subgroup of EnOC harbouring MMRm, with a similar overall MMRm rate as reported previously in EnOC [30] , [31] , [32] , [33] , [34] . We demonstrate that cases with high impact MMRm (nonsense, frameshifting or splice site mutations) demonstrate MSI and that these cases account for many of the samples demonstrating high TMB. POLE m was rare in this cohort (6.3% of cases); there was significant enrichment for MMRm within this population ( P = 0.002) and concurrent mutation of POLE and MMR genes was present in all three ultramutated tumours. Notably, when considering only missense MMRm, we observed no significant difference in MSI score compared to MMRwt cases, suggesting fewer missense mutations lead to functional loss of MMR. Moreover, POLE m cases did not appear to demonstrate the exceptional 5-year survival reported in POLE m endometrial carcinomas [11] , and was not associated with significantly prolonged survival, though the power of this analysis was severely limited. The low POLE m rate we observed is consistent with previous reports in EnOC [35] , [36] . Collectively, the data presented here identify TP53 m EnOC as a distinct clinical and biological subtype of disease. TP53 m cases demonstrated higher levels of CNA events, greater tumour genomic complexity, higher rate of advanced stage at diagnosis, inferior rate of complete macroscopic tumour resection, and overall poor clinical outcome. This is consistent with the poor prognosis reported in EnEC harbouring TP53 m [11] , is reminiscent of HGSOC [12] , and is in line with several studies of EnOC [28] , [37] . In particular, the study performed by Parra-Herran et al. [28] applied the PROMISE algorithm, an EnEC molecular classifier, to a cohort of WT1 negative EnOC and found the p53-aberrant group to have the worst survival; a recent study of early stage EnOC also reported poor outcome for cases with p53-aberrant cases [38] . In our cohort, TP53 m cases also represented those least likely to demonstrate concurrent endometrial cancer. While the copy number and survival profile of our TP53 m EnOC group provides one rationale for reclassification of these tumours as HGSOC, the high frequency (48.3%, 14 of 29) of classic EnOC mutations ( CTNNB1 , PTEN , ARID1A , KRAS, PIK3CA , or MMRm), lack of WT1 expression (in all cases) and high rate of early stage diagnosis in this cohort (51.7%, 15 stage I/II) form a compelling argument that these represent true EnOC. Indeed, these poorer prognosis EnOC cases may well be suitable for inclusion alongside true HGSOC in trials of novel therapeutic strategies for aggressive OC types. Only nine cases (8.0% of our cohort) represented feasible candidates as possible true WT1-negative HGSOC (advanced stage at diagnosis and TP53 m without mutations suggestive of endometrioid carcinoma i.e., MMR, PTEN , CTNNB1 , PIK3CA , ARID1A and KRAS wild-type), which are recognised as a rare phenomenon (≤5% HGSOC cases) [24] . The true histological subtype of this small group cannot be determined with absolute certainty; however, sensitivity analysis excluding possible occult serous carcinomas of ovarian or endometrial origin identified the same outcome differences between genomic subtypes. Conversely, CTNNB1 m—which appears mutually exclusive with TP53 m—is associated with early-stage disease of low genomic complexity that is easily debulked to zero macroscopic RD, and these cases demonstrate excellent clinical outcome. This is in contrast to findings in EnEC associating CTNNB1 m with a greater chance of recurrence [39] . Within our EnOC cohort, CTNNB1 m status was also associated with favourable outcome specifically in the context of TP53 wt tumours, suggesting clinical impact independent of its anti-correlation with TP53 m. These data support the notion of a tiered classification system driven by TP53 m and CTNNB1 m status to define molecular subtypes of EnOC with markedly differential clinical outcome and clinicopathological features; this classifier—the PRISTINE algorithm—should now be validated in an independently curated, sufficiently powered EnOC dataset defined using contemporary criteria, including the use of WT1 IHC. We demonstrate that consideration of genomic complexity may provide a potential future way to further resolve outcomes within these subgroups, though this analysis was exploratory in nature. Despite the variability in processing, age, fixation and preservation of tissue specimens, we demonstrate that IHC for p53 and β-catenin proteins can recapitulate this classification system, but is limited by the sensitivity of β-catenin IHC for detecting CTNNB1 m, consistent with previous reports of β-catenin immunostaining as a surrogate for CTNNB1 m [40] , [41] . Implementation of IHC-based classification may well demonstrate improved sensitivity/specificity in newly diagnosed cases with uniformly fixed, well preserved whole-slide tissue sections. The high rate of genomic disruption in CTNNB1 , KRAS , PTEN and PIK3CA suggests that inhibitors of the WNT, MAPK and PI3K pathways represent agents with potential clinical utility in EnOC treatment. Efforts to identify novel therapeutic strategies should focus on cases with greatest unmet clinical need, namely CTNNB1 wt cases. In particular, TP53 m cases represent those where further treatment options are urgently required to improve outcome, and we identified potentially clinically actionable mutations in a large proportion of these cases (14% with KRAS m, 28% with PTEN m/ PIK3CA m, 28% with BRCA1/2 m). Finally, we identify SOX8 as a gene target of recurrent mutation in EnOC. SRY-related high mobility group box ( SOX ) genes encode a family of transcription factors, which act as critical regulators of cellular programming and are frequently altered in many cancers [42] . Interestingly, analysis of TCGA data reveals that SOX8 m occurs at low frequency in uterine cancers (3% in uterine corpus endometrial carcinoma, 1% in uterine carcinosarcoma) as well as in colonic adenocarcinoma (2%) (data from the TCGA portal [43] ). As recent studies suggest that SOX8 in part regulates the activity of genes associated with the WNT/β-catenin pathway, a commonly mutated pathway in EnOC, mutation of this gene may impact on classically defined EnOC pathways through this route [44] . Genomic disruption of SOX8 therefore represents a previously unreported candidate mechanism by which EnOC may frequently perturb the WNT/β-catenin pathway. Given the frequent co-occurrence of SOX8 m and TP53 m in our cohort (34.5% SOX8 m in the TP53 m group), selection bias against true high grade EnOC in previous studies—leading to depletion of TP53 m cases in those cohorts—may explain why SOX8 m has not previously been identified as a common genomic event in EnOC. Beyond genomic characterisation, a transcriptomic study of EnOC identified clinically meaningful patient subgroups defined at the gene expression level akin to those previously described in HGSOC [18] . Interestingly, while the poorer prognosis of genomically complex EnOC cases we describe here might be expected to produce a more pronounced anti-tumour immune response, the immunoreactive transcriptomic subgroup they identified did not demonstrate the poorest outcome. Future work should seek to correlate EnOC subgroups defined at these different levels in order to determine the association between genomic and transcriptomic events in this tumour type. Similarly, comparison with subgroups defined at the proteomic level, including those based on expression patterns of hormone receptors [45] , should be made. In summary, we have demonstrated that EnOC is a molecularly heterogeneous disease, comprising multiple genomic subtypes. These subtypes demonstrate differential clinical outcome and clinicopathological features. In particular, our study highlights CTNNB1 m and TP53 m as markers of biologically distinct subtypes of EnOC with contrasting clinical behaviour. These markers have the potential to inform future prognostication and molecular stratification within EnOC. Gene sequencing of TP53 and CTNNB1 , or IHC directed at their respective gene products, represent mechanisms by which these findings could readily be translated into routine risk-stratification of newly diagnosed cases. Patients with EnOC demonstrating absence of CTNNB1 m and/or presence of TP53 m have the greatest unmet clinical need; many of these tumours harbour activating mutations in pathways that may be targetable with molecular agents. Investigating the clinical efficacy of inhibitors of the MAPK/RAS, WNT and PI3K pathways has the potential to identify agents that will improve EnOC patient survival. Ethical approval Ethical approval for the use of human tissue specimens for research was obtained from South East Scotland Scottish Academic Health Sciences Collaboration BioResource (reference 15/ES/0094-SR494). Correlation of molecular data to clinical outcome and clinicopathological variables in ovarian cancer was approved by NHS Lothian Research and Development (reference 2007/W/ON/29). All relevant ethical regulations have been complied with, including the need for written informed consent where required. Pathology review and immunohistochemistry 505 patients diagnosed with OC between August 1968 and May 2014, and whose pathology reports contained the term “endometrioid”, were identified through the Edinburgh Ovarian Cancer Database (Fig. 1 ); tumour material was available for 289 cases [45] . Chemotherapy naïve tumour from the primary site was selected where available. Pathology review was conducted as per WHO 2014 classification, including IHC for WT1 in every case (see Supplementary Methods ), by an expert gynaecological pathologist (CSH). A confirmatory observer (BS) was present for all pathology review. The presence of endometriosis was recorded from the reviewed slides or pathology report. Cases with non-interpretable morphology, non-evaluable tumour and cases representing metastases from primary endometrial cancer, as defined by WHO criteria, were excluded. Ovarian metastases, WT1 positive tumours, carcinosarcomas and carcinomas of clear cell, mucinous or mixed histology were also excluded (Fig. 1 ). IHC for cytokeratin 7 and cytokeratin 20 (CK7 and CK20) was performed to exclude colorectal adenocarcinoma metastases (see Supplementary Methods ). p53 and β-catenin IHC was performed as described in the Supplementary Methods . Clinical data Baseline characteristics and outcome data were extracted from the Edinburgh Ovarian Cancer Database, wherein the diagnostic, treatment and follow-up data for every ovarian cancer patient treated at the Edinburgh Cancer Centre is prospectively entered as a part of routine care [5] . DSS was calculated from the date of pathologically confirmed OC diagnosis. PFS was recorded as the duration between the date of diagnosis to the date of first radiological progression or recurrence, or death from EnOC. DNA extraction H&E-stained slides were marked by an expert gynaecological pathologist (CSH) to identify tumour areas suitable for macrodissection in order to enrich for tumour cellularity. DNA extraction was performed using the QIAamp DNA formalin-fixed paraffin-embedded (FFPE) Tissue Kit (Qiagen, Venlo, Netherlands) and Deparaffinization Solution according to the manufacturer’s instructions. Whole exome sequencing Exome capture was performed using the Illumina TruSeq Exome Library Prep kit (see Supplementary Methods ) and WES was performed on the Illumina NextSeq 550 (Illumina, Inc., San Diego, CA, USA). The median per-sample on-target coverage in the successfully sequenced samples was 89.5× (range 36×–289×). Data were aligned to the GRCh38 human reference genome using bwa-0.7.17 [46] , duplicates marked and base quality scores recalibrated with the GenomeAnalysisToolkit (GATK) v4 [47] in the bcbio pipeline (see Supplementary Methods ). Variant calling and classification Variant calling was performed using a majority vote system from three variant caller algorithms: VarDict [48] , Mutect2 [49] and Freebayes [50] . Filtering for FFPE and oxidation artifacts was applied using GATK CollectSequencingArtifactMetrics and FilterByOrientationBias. Variants associated with low sequence depth (<20×) or low variant allele frequency (<10%) were removed. Common variants were excluded using the 1000 genomes and ExAC reference datasets; known pathogenic and benign variants were flagged using ClinVar [51] , and remaining variants were filtered to remove likely non-functional variation using the Polymorphism Phenotyping (PolyPhen) [52] and Sorting Intolerant from Tolerant [53] functional prediction tools (see Supplementary Methods ). MSI score was assessed as the number of short insertions or deletions (InDels) detected in a given sample. TMB was defined as the number of mutations present in a given tumour following filtering. TMB across other cancer datasets in The Cancer Genome Atlas (TCGA) were contrasted against those in our EnOC datasets [54] . Transitions and transversions were calculated using the titv function in maftools [55] . Unsupervised analysis was performed using the top 50 most frequently mutated genes represented as a binary matrix (0, wild-type; 1, mutant). Product-moment correlation scores were calculated between these binary signatures of each sample to form a matrix of quantified genomic correlation. Samples were then clustered by Euclidian distance and Ward’s linkage based on this correlation matrix. Heat maps were drawn in R using the ggplot package. Supervised mutational analysis was performed using the most commonly mutated genes across sequenced samples. Genomic events in these genes and overall TMB analysis were visualised using the R package maftools [55] . Pathway analysis was carried out using the OncogenicPathways function [56] . Tumour genomic complexity scoring Tumour genomic complexity was assessed by VAF density using the inferHeterogeneity function in the R package maftools [55] , [57] (see Supplementary Methods ). Resulting MATH scores represent the width of the VAF distribution; specimens of low complexity with a single driver event and associated outgrowth demonstrate fewer VAF peaks with a lower MATH score. Conversely, highly complex tumours with multiple driver events, branched evolution and multiple subclonal populations demonstrate multiple VAF peaks and higher MATH score. Copy number alteration detection Copy number analysis was performed using GeneCN pipelines in Bio-DB-HTS version 2.10 to identify regions of significant copy number gain or loss (copy number score >5 standard deviations from reference, P < 0.05) using the pooled TP53 wt samples as a reference population. Statistical analysis Statistical analyses were performed using R version 4.0.0. Comparisons of continuous data were made with the Mann–Whitney U -test or T -test, as appropriate. Median follow-up time was calculated using the reverse Kaplan–Meier method. Survival analysis was performed using Cox proportional hazards regression models in the Survival package. Multivariable analyses accounted for FIGO stage, patient age at diagnosis, decade of patient diagnosis and extent of RD following surgical cytoreduction. Comparisons of frequency were performed using the Chi-square test or Fisher’s exact test, as appropriate. Correction for multiplicity of testing was performed using the Bonferroni method where appropriate. Reporting summary Further information on research design is available in the Nature Research Reporting Summary linked to this article.